CaV1.3-selective L-type calcium channel antagonists as potential new therapeutics for Parkinson's disease L-type calcium channels expressed in the brain are heterogeneous. The predominant class of L-type calcium channels has a Ca V 1.2 pore-forming subunit. L-type calcium channels with a Ca V 1.3 pore-forming subunit are much less abundant, but have been implicated in the generation of mitochondrial oxidant stress underlying pathogenesis in Parkinson's disease. Thus, selectively antagonizing Ca V 1.3 L-type calcium channels could provide a means of diminishing cell loss in Parkinson's disease without producing side effects accompanying general antagonism of L-type calcium channels. However, there are no known selective antagonists of Ca V 1.3 L-type calcium channel. Here we report high-throughput screening of commercial and 'in-house' chemical libraries and modification of promising hits. Pyrimidine-2,4,6-triones were identified as a potential scaffold; structure-activity relationship-based modification of this scaffold led to 1-(3-chlorophenethyl)-3-cyclopentylpyrimidine-2,4,6-(1 H ,3 H ,5 H )-trione ( 8 ), a potent and highly selective Ca V 1.3 L-type calcium channel antagonist. The biological relevance was confirmed by whole-cell patch-clamp electrophysiology. These studies describe the first highly selective Ca V 1.3 L-type calcium channel antagonist and point to a novel therapeutic strategy for Parkinson's disease. Parkinson's disease (PD) is the most common neurodegenerative movement disorder, characterized by tremors, bradykinesia and rigidity [1] . PD has no cure, and nothing is known to slow its progression. The defining motor symptoms of PD result from the degeneration of dopaminergic neurons in the substantia nigra pars compacta (SNc) [2] , [3] . Recently, we reported that the engagement of L-type calcium channels [4] (LTCCs) during autonomous pacemaking renders adult SNc neurons vulnerable to toxins used to create models of PD [5] . More recently, we demonstrated that the activity-dependent engagement of LTCCs elevates mitochondrial oxidant stress in SNc dopaminergic neurons, providing a means by which LTCCs could increase toxin sensitivity [6] . Interestingly, LTCCs do not appear to be necessary for normal functioning of SNc dopaminergic neurons, making them viable therapeutic targets [7] . The involvement of LTCCs in determining neuronal vulnerability is based on the ability of 1,4-dihydropyridines [8] (DHP) to protect SNc dopaminergic neurons against toxins and to diminish their mitochondrial oxidant stress. DHPs are use-dependent antagonists of LTCCs that have a long history of success in the treatment of hypertension in humans [9] . In agreement with the propositions that LTCCs contribute to pathogenesis, retrospective epidemiological studies conducted in the United Kingdom [10] and Denmark [11] have revealed that the treatment of hypertension with DHPs that cross the blood–brain barrier diminish the observed risk of PD. The problem with DHPs from a therapeutic perspective, however, is that they are not selective [12] . LTCCs are a heterogenous class of multi-subunit ion channels [13] , [14] that can be divided into four classes based on the identity of their pore-forming alpha 1 subunit, Ca V 1.1-4. This pore-forming subunit governs key features of the channel, including gating and pharmacology. The predominant (~90%) LTCC in the brain has a Ca V 1.2 subunit; this channel also is abundant in a variety of peripheral organ systems, including the cardiovascular system and is effectively antagonized by DHPs, accounting for their therapeutic efficacy in hypertension [15] . However, the LTCC responsible for mitochondrial oxidant stress and increased vulnerability in SNc dopaminergic neurons is largely attributable to expression of LTCCs with a Ca V 1.3 subunit [5] , [6] . Among the DHPs, isradipine has the highest relative affinity for Ca V 1.3 LTCCs, but it is still Ca V 1.2 LTCC selective [14] . This diminishes the therapeutic potential of DHPs in PD, as cardiovascular side effects limit the dosing and antagonism of Ca V 1.3 LTCCs. As there are no selective Ca V 1.3 LTCC antagonists known, there is a real translational need to develop a new therapeutic agent. The antagonistic effects of well-known LTCC antagonists [16] , [17] , like isradipine, verapamil and diltiazem ( Fig. 1a ), were investigated with stably expressing Ca V 1.3 and Ca V 1.2 LTCCs in HEK293 cells. Using a fluorometric imaging plate reader (FLIPR) [18] assay with Fluo-8 calcium dye [19] , we found that all three were weak antagonists of Ca V 1.3 LTCCs, and all were more potent antagonists of Ca V 1.2 LTCCs. Over 100 DHPs were screened in an attempt to identify a Ca V 1.3 channel selective antagonist [20] ; however, none was selective for Ca V 1.3 LTCCs. As a consequence, a screen of novel small molecules was undertaken, and the Ca V 1.3-selective hits were modified. Here we report the identification of the first highly selective Ca V 1.3 LTCC antagonist ( 8 ). 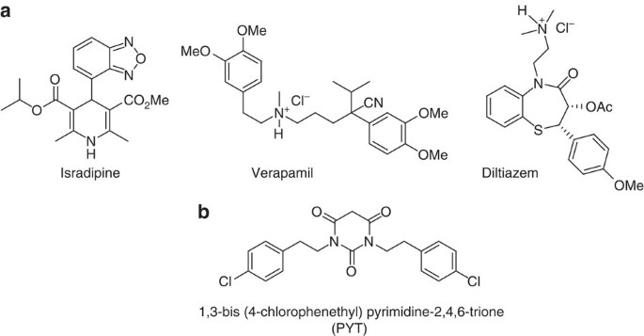Figure 1: Various LTCC antagonists. (a) Antihypertensive drugs that non-selectively antagonize LTCCs (b) HTS initial hit compound PYT. Figure 1: Various LTCC antagonists. ( a ) Antihypertensive drugs that non-selectively antagonize LTCCs ( b ) HTS initial hit compound PYT. Full size image High-throughput screen setup and identification of hits The biological assay utilized a preparation of HEK293 cells that stably expressed Ca V 1.3 and Ca V 1.2 LTCCs. A FLIPR-based high-throughput screen (HTS) for both Ca V 1.2 and Ca V 1.3 LTCCs was used to screen 60,480 commercial compounds (ADSI set of 6,800 compounds; ChemBridge diverse/lead like set of 20,000 compounds; ChemDiv diverse set of 30,000 compounds; NIH clinical trial set of 480 compounds and NCI/DTP set of 3,200 compounds (see the DTP website address http://dtp.cancer.gov (2012)). Testing of these commercial compounds for Ca V 1.3 LTCCs resulted in not a single hit. Subsequently, we screened a few hundred compounds from our (Silverman lab) non-commercial compound library. From that screen, the pyrimidine 2,4,6-trione (PYT) scaffold was identified as the first class of selective antagonists for Ca V 1.3 LTCCs. The initial symmetric PYT hit ( Fig. 1b ) displayed moderate potency and Ca V 1.3 channel selectivity (approximately eightfold from a comparison of the IC 50 value with Ca V 1.3 to that with Ca V 1.2). The scaffold also was of interest because of its favourable pharmacological and absorption, distribution, metabolism and excretion (ADME) properties, as well as low toxicity, brain penetration and oral bioavailability, as previously determined [21] . Structure-activity relationship-based hit modification About 120 PYT analogues were synthesized to develop insight into structure-activity relationships (SARs). The general approach taken to N,N -disubstituted PYT synthesis involved the use of the Wöhler [22] urea synthesis, the coupling of isocyanate with various amines, and Biltz and Wittek's [23] condensation of ureas with activated malonic acid ( Fig. 2 ). Treatment of malonyl chloride with the ureas provided the condensation products in good yields. Further optimization of each step allowed a one-pot parallel synthesis, and sufficient sample purity was achieved by fractional filtration of the final reaction mixture through a silica gel plug (10 cm). This synthetic route permitted the construction of the majority of the PYT library members in sufficient quantities and purity for assay against Ca V 1.3 and Ca V 1.2 LTCCs; promising compounds were purified further and retested. 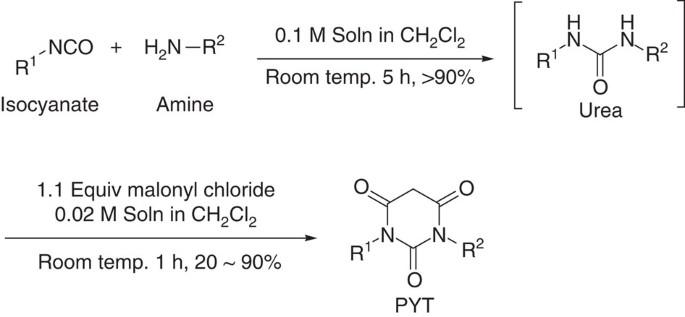Figure 2: Common synthetic route to the PYT scaffold. Procedures are described in detail in Methods and inSupplementary Methods, and characterization of the compounds is given inSupplementary Methods. Figure 2: Common synthetic route to the PYT scaffold. Procedures are described in detail in Methods and in Supplementary Methods , and characterization of the compounds is given in Supplementary Methods . Full size image Using this methodology three sets of PYT analogues were synthesized to probe different structural features of the initial hit PYTs, including substitutions on each of the nitrogens of the PYT core ( Fig. 3 ). The results of the assay are shown in Table 1 . The trend that emerged from this library was a steric effect of the lipophilic side chain. Among the cycloalkyl groups, the cyclopentyl derivatives ( 7 and 8 ) were the most highly selective antagonists for the Ca V 1.3 LTCCs; 8 (1-(3-chlorophenethyl)-3-cyclopentylpyrimidine-2,4,6-(1 H ,3 H ,5 H )-trione) was the most isoform-selective Ca V 1.3 antagonist, inhibiting Ca V 1.3 LTCCs >600-fold more potently than Ca V 1.2 LTCCs, (determined from the ratio of IC 50 values) with an IC 50 of 1.7 μM ( Fig. 4 ). Compounds 9 and 10 were the most potent antagonists of this series of molecules (800 nM and 600 nM, respectively), having moderate selectivity (~25-fold). 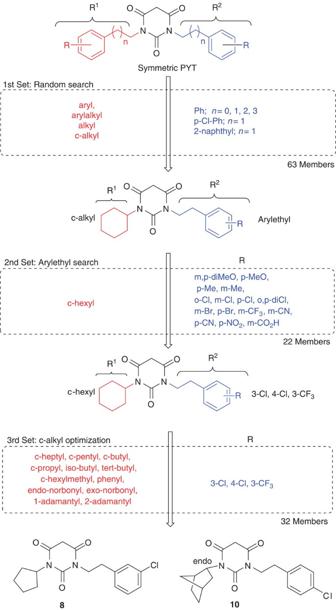Figure 3: General scheme for SAR-based modifications. Three regions of structural modifications are defined with the number of compounds prepared in each set to interrogate those regions. Figure 3: General scheme for SAR-based modifications. Three regions of structural modifications are defined with the number of compounds prepared in each set to interrogate those regions. Full size image Table 1 IC 50 values and selectivity of select PYT analogues after lead modification. 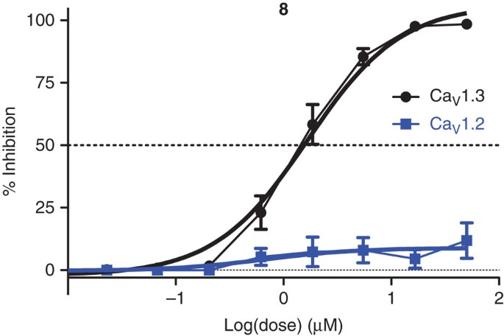Figure 4: Concentration-dependent LTCC antagonism by8in FLIPR assay. FLIPR assay concentration dependence of percentage inhibition for CaV1.3 LTCCs and CaV1.2 LTCCs with compound8. Curves are drawn with nonlinear regression (mean±s.e.m.) using Prism. CaV1.3: IC50=1.7±0.2 μM; CaV1.2: IC50=not observed (calculated IC50=1730±469 μM). Values are mean±s.d.;n=6 for both CaV1.3 and CaV1.2. The values are measured by sigmoidal fit using XLfit. Full size table Figure 4: Concentration-dependent LTCC antagonism by 8 in FLIPR assay. FLIPR assay concentration dependence of percentage inhibition for Ca V 1.3 LTCCs and Ca V 1.2 LTCCs with compound 8 . Curves are drawn with nonlinear regression (mean±s.e.m.) using Prism. Ca V 1.3: IC 50 =1.7±0.2 μM; Ca V 1.2: IC 50 =not observed (calculated IC 50 =1730±469 μM). Values are mean±s.d. ; n =6 for both Ca V 1.3 and Ca V 1.2. The values are measured by sigmoidal fit using XLfit. Full size image Pharmacophoric model The crystallographic data of 8 are given in a .cif file ( Supplementary Data 1 ) and are available from the Cambridge Crystallographic Data Centre (deposition number CCDC 899840). Crystal data for 8 : Monoclinic, Pn space group, a =6.9749(2) Å, b =30.6660(8) Å, c =7.3929(2) Å, β =92.0160(10)°, V =1580.31(7) Å 3 , Z =4, R 1 =0.0329, wR 2 =0.0861, F.W.=334.79, c.d.=1.407 g cm −3 . X-ray crystallographic analysis of compound 8 shows that the PYT ring is oriented perpendicularly to the plane of the cycloalkyl ring ( Fig. 5 ). As the most selective PYTs have an N -substituted cycloalkyl group, it is possible that the Ca V 1.3 channel can accommodate a PYT ring twisted relative to the plane of the N -cycloalkyl group, but the Ca V 1.2 channel cannot. 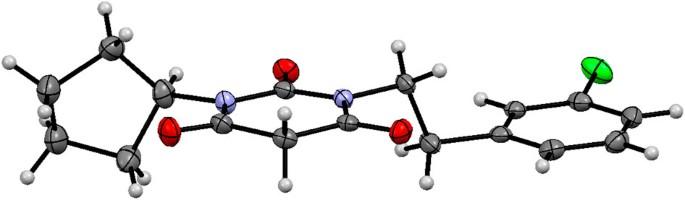Figure 5: X-ray crystal structure of compound8. The cyclopentyl ring is perpendicular to the PYT ring (CCDC deposition number 899840). Figure 5: X-ray crystal structure of compound 8 . The cyclopentyl ring is perpendicular to the PYT ring (CCDC deposition number 899840). Full size image Bioactivity and relevance confirmation As IC 50 values determined in our FLIPR assay depend strongly on assay conditions, the absolute values and selectivity patterns attained through this assay were confirmed using a technically different, yet relevant, measure. To that end, the inhibition of stably expressing Ca V 1.3 and Ca V 1.2 LTCCs by compound 8 was measured by voltage-clamp experiments ( Fig. 6 ). Whole-cell voltage-clamp recordings ( Fig. 6a,b ) in the presence of compound 8 showed that 8 selectively (as determined by the ratio of Ca V 1.3 to Ca V 1.2 inhibition by 8 at a given concentration) inhibits Ca V 1.3 LTCCs over Ca V 1.2 LTCCs. Compound 8 at 5 μM exhibited 31.2% and 4.4% inhibition for Ca V 1.3 and Ca V 1.2 channel current, respectively ( Fig. 5c ), which correlates with the results of the FLIPR assay (85.4% and 8.0% inhibition for Ca V 1.3 and Ca V 1.2 LTCCs, respectively, at 5.5 μM concentration). The observed IC 50 with 8 for Ca V 1.3 from the whole-cell patch clamp experiment was 24.3±0.7 μM, and because the potency of 8 was too small to generate a concentration–response curve for Ca V 1.2 channels, the IC 50 with 8 for Ca V 1.2 was not computed. 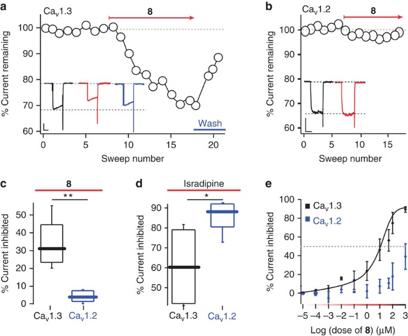Figure 6: Whole-cell patch-clamp experiments. Time course of effects of (a) CaV1.3 and (b) CaV1.2 calcium channel peak currents (○) for compound8(5 μM). Example of current traces from control (black), compound8(red), and wash (blue) are inserted. All vertical scale bars are 50 pA, and horizontal scale bars are 50 ms. Population data of the inhibition conferred by (c), compound8(5 μM) with CaV1.3 (black,n=17, median=0.312) and CaV1.2 (blue,n=10, median=0.0439), which was deemed signficant by the Mann–Whittney rank-sum Test (**P<0.001); and (d), isradipine (300 nM) with CaV1.3 (black,n=5, median=0.604) and CaV1.2 (blue,n=5, median=0.881), which was deemed significant by the Mann–Whittney Ram-sum test (*P<0.05). (e) Concentration–response curves for compound8inhibition of CaV1.3 and CaV1.2 LTCCs. Data were fit to the Hill equation: (Icontrol−Icompound8)/Icontrol=1/(1+(IC50/Ccompound8)h), where IC50is the concentration of compound8required to inhibit 50% of peak current, andhis the Hill cofficient. CaV1.3: IC50=24.3±0.7 μM;h=0.42±0.04; CaV1.2: IC50=not observed;h=not observed. Figure 6: Whole-cell patch-clamp experiments. Time course of effects of ( a ) Ca V 1.3 and ( b ) Ca V 1.2 calcium channel peak currents ( ○ ) for compound 8 (5 μM). Example of current traces from control (black), compound 8 (red), and wash (blue) are inserted. All vertical scale bars are 50 pA, and horizontal scale bars are 50 ms. Population data of the inhibition conferred by ( c ), compound 8 (5 μM) with Ca V 1.3 (black, n =17, median=0.312) and Ca V 1.2 (blue, n =10, median=0.0439), which was deemed signficant by the Mann–Whittney rank-sum Test (** P <0.001); and ( d ), isradipine (300 nM) with Ca V 1.3 (black, n =5, median=0.604) and Ca V 1.2 (blue, n =5, median=0.881), which was deemed significant by the Mann–Whittney Ram-sum test (* P <0.05). ( e ) Concentration–response curves for compound 8 inhibition of Ca V 1.3 and Ca V 1.2 LTCCs. Data were fit to the Hill equation: ( I control − I compound 8 )/ I control =1/(1+(IC 50 / C compound 8 ) h ), where IC 50 is the concentration of compound 8 required to inhibit 50% of peak current, and h is the Hill cofficient. Ca V 1.3: IC 50 =24.3±0.7 μM; h =0.42±0.04; Ca V 1.2: IC 50 =not observed; h =not observed. Full size image As Ca V 1. 3 and Ca V 1.2 LTCC-expressing cells were used for comparative screens, it was necessary for each of these cell lines to have similar characteristics to allow ready comparison of compound activity. To this end, cell lines with roughly equivalent channel densities were grown, aliquoted and then cryopreserved, so that the cells used for the assay remained homogenous throughout the screening process. Compounds selected for this screen were not from libraries containing known ion channel antagonists because we wanted to identify novel molecules that were not only selective for Ca V 1.3 LTCCs, but also were unlikely to significantly antagonize other classes of ion channels. The first library of PYTs (63 members) was synthesized to probe several different structural features based on results from our initial hit PYTs, including substitution on the side chain and substitution on the aryl ring ( Fig. 3 ). Four R 2 substituents were used (4-chlorophenethyl, 3-phenylpropyl, 4-phenylbutyl and 2-naphthylethyl). To probe the electronic effects and steric demands on the R 1 aryl ring, electron-withdrawing (F, Cl, Br, CF 3 and NO 2 ) substituents and methyl were chosen. As electron-rich substituents in the original library did not exhibit good selectivity or potency with Ca V 1.3 LTCCs, electron-rich substituents (except methyl) were not considered at this stage. To probe the required distance between the PYT ring and the aryl ring of R 2 , four different alkyl chains (C 1 –C 4 ) were incorporated into the sidechain. To probe the steric requirements of R 1 , cyclopentyl, cyclohexyl, 2-phenylpropyl, indanyl and tetralinyl substituents were used. From the first library of analogues assayed, three members ( 1 , 2 and 3 ) were shown to inhibit Ca V 1.3 LTCCs with excellent selectivity (>28-fold from a comparison of the IC 50 value with Ca V 1.2 to that with Ca V 1.3) compared with that of the initial hit ( Table 1 ). This is the first class of antagonists that inhibits Ca V 1.3 considerably more potently than Ca V 1.2 LTCCs. The bulky R 1 cycloalkyl group may be involved in specific steric interactions with neighbouring residues in the Ca V 1.2 channel-binding site causing weak binding. All of the analogues assayed, and their associated activities, are shown in Supplementary Tables S1–S3 . The second library (22 members) was prepared to probe the electronic and steric demands on aryl ring R 2 using a cyclohexyl group for R 1 . Electron-withdrawing substituents (F, Cl, Br, CF 3 , CO 2 H, CN and NO 2 ) and electron-donating substituents (MeO, Me) were used on the R 2 side ( Fig. 3 ). When R 1 was cyclohexyl, the analogues with R 2 m -chlorophenethyl ( 3 ), m -methylphenethyl ( 4 ), m -bromophenethyl ( 5 ) and m -trifluoromethylphenethyl ( 6 ) were the most selective antagonists for Ca V 1.3 LTCCs ( Table 1 ). The selectivity of the meta-substituted analogues results from the loss of antagonism to Ca V 1.2 LTCCs. This meta-substitution effect also prevailed when utilizing cyclopentyl as the R 1 substituent, encompassing the third library. However, hydrophilic functional groups on the arylalkyl R 2 diminished antagonism to both LTCCs; -CO 2 H, -NO 2 , -CN or -OMe substituted arylalkyl members mostly displayed IC 50 values >9 μM for both Ca V 1.3 and Ca V 1.2 LTCCs. The third library (32 members) was prepared to probe the steric demands on R 1 , while maintaining the three best side chains ( m -chlorophenethyl, p -chlorophenethyl and m -trifluoromethylphenylethyl) of previous libraries as R 2 . Cycloalkyl substituents (cycloheptyl, cyclohexyl, cyclopentyl, cyclobutyl and cyclopropyl), bicycloalkyl substituents ((±)-2- endo -norbonyl, (±)-2- exo -norbonyl), tricycloalkyl substituents (1-adamantyl, 2-adamantyl), and various other bulky substituents were used for R 1 ( Fig. 3 ). Three general pharmacophores can be drawn after analysing all of the trends. First, the most selective compounds for Ca V 1.3 LTCCs have a cyclohexyl or cyclopentyl substituent (R 1 ) on the PYT skeleton, implying that a perpendicularly arranged 5- or 6-membered alkyl ring is needed for selective antagonism of the Ca V 1.3 LTCCs. Second, a meta-substituted phenethyl moiety (R 2 ) improves selectivity for the Ca V 1.3 LTCCs. Third, Ca V 1.3 LTCCs respond to a variety of bulky structures at the cycloalkyl binding site; however, substituents with exceptional steric demand antagonize non-selectively. HEK293 cells that stably expressed Ca V 1.3 and Ca V 1.2 LTCCs using the FLIPR assay ( Fig. 4 ) and whole-cell voltage-clamp recordings ( Fig. 6 ) confirmed the Ca V 1.3 selectivity of 8 . Although the two assay methods and relative magnitude of inhibition of 8 are different; the observed % of inhibition and IC 50 values confirm that PYT is a viable selective antagonist scaffold, and compound 8 is a highly selective analogue. In conclusion, Ca V 1.3 LTCCs have recently been implicated in the pathogenesis of PD; however, there are no known selective antagonists for Ca V 1.3 LTCCs. To address this important medical need, a HTS using a FLIPR calcium assay was performed on diverse chemical libraries as an attempt to identify Ca V 1.3-selective antagonists. The PYT scaffold was identified, and further SAR based modifications led to 1-(3-chlorophenethyl)-3-cyclopentylpyrimidine-2,4,6-(1 H ,3 H ,5 H )-trione ( 8 ), the first potent and highly selective Ca V 1.3 antagonist, confirmed by whole-cell voltage-clamp recordings of HEK293 cells expressing functional Ca V 1.3 and Ca V 1.2 LTCCs. This novel compound is undergoing preclinical evaluation. Transfection of HEK293 cells with Ca V 1. 3 and Ca V 1.2 Rat Ca V 1.3α1D (GenBank accession number: AF370010 ) containing all alternative splice sites, rat Ca V β3 (GenBank accession number: M88751 ), rat Ca V α2δ-1 (GenBank accession number: AF286488 ) and rabbit Ca V 1.2α1C (GenBank accession number: P15381 ) complementary DNAs were used. The potential difference in drug sensitivity caused by alternative splice isoforms of either Ca V 1.2 or Ca V 1.3 were not evaluated in these studies. All constructs were provided by Dr Diane Lipscombe (Brown University) and Dr Johannes Hell (University of Iowa). General methods for constructs development and transfection [14] , [20] of Ca V 1.2α1C or Ca V 1.3α1D, Ca V β3 and Ca V α2δ-1 into HEK293 cells for FLIPR screens were described in our earlier study [20] . General procedure for high-throughput screening Ca V 1.3. or Ca V 1.2 LTCCs antagonism was determined using Screen Quest Fluo-8 NW Calcium Assay Kit (ABD Bioquest Inc., Sunnyvale, CA, USA) on a FLIPR tetra (Molecular Devices LLC, Sunnyvale, CA, USA) as follows: HEK293 cells (4×10 4 cells per well) expressing either Ca V 1.2 or Ca V 1.3 LTCCs were cultured in DMEM with 10% fetal bovine serum for 4 days on tissue culture-treated, 384-well plates, clear-bottom black plates (Greiner Bio-One North America Inc., Monroe, NC, USA). The assay plates were coated with BD Matrigel matrix to improve cell adherence. Dilution series of lead compounds were generated in separate 384-well plates using an Echo550 acoustic liquid transfer system (Labcyte Inc., Sunnyvale, CA, USA). Fluo-8 reagent was prepared in Hanks-buffered saline solution(+) (with 20 mM Hepes and 5 mM additional CaCl 2 added, pH 7.4). Then 100 μl of the Fluo-8 reagent was added to the compound dilution series and controls, and well mixed by pipetting using a Biomek FX liquid handler (Beckman Coulter Inc., Brea, CA, USA). The media was then removed from the cells and 45 μl of the compound/Fluo-8 mixture was transferred to assay plates of each cell line using the Biomek FX. The treated cells were incubated at 37 °C for 45 min and then removed from the incubator and placed at room temperature for an additional 30 min. The plates were placed in the FLIPR tetra, which was programmed to measure the fluorescence intensity before, during and for 2 min after adding 25 μl of KCl solution (450 mM KCl in Hanks-buffered saline solution(+) solution, pH 7.4). FLIPR tetra data acquisition parameters were as follows: excitation wavelength 470–495 nm, emission wavelength 515–575 nm, gain 80, exposure 0.4 s, excitation intensity 80. General procedure for whole-cell patch-clamp assay After 24–48 h of incubation at 37 °C on poly- D -lysine-treated coverslips, stably transfected HEK293 cells underwent whole-cell patch-clamp electrophysiology. The external solution contained the following (in mM): 140 NaCl, 1 MgCl 2 , 10 BaCl 2 , 10 HEPES, 10 dextrose, 10 sucrose and 20 CsCl at pH 7.4 and an osmolarity of ~320 mOSm l −1 . The test compound stock solutions in dimethylsulphoxide (100 mM or just dimethylsulphoxide) were diluted with the external solution to the desired concentration (10 −9 to 10 −3 M), which was perfused (2 ml per min) into the recording chamber while measuring the evoked barium currents. In experiments where concentration–response curves were obtained, local perfusion of the desired concentration was employed. Barium currents were measured from whole-cell voltage patch-clamp recordings using the Pulse 8.4 software data acquisition system (HEKA, Germany). Signals were low-pass filtered at 1 kHz, digitized (sampled) at 10 kHz, and were amplified with an Axopatch 200B patch-clamp amplifier (Axon Instruments). Barium currents were evoked by a depolarizing voltage step from a holding potential of −70 to 0 mV for 100 ms with a frequency of 0.05 Hz at room temperature (22–25 °C). Patch pipettes were pulled from thin-wall borosilicate glass coated with dental wax and maintained at a resistance of ~3–5 mΩ. Internal pipette solutions contained the following (in mM): 180 N -methyl- D -glucosamine, 40 HEPES, 4 MgCl 2 , 12 phosphocreatine, 0.1 leupeptin, 2 Na 2 ATP, 0.5 Na 3 GTP, 5 BAPTA, pH 7.2–7.3 and an osmolarity of ~290 mOSm l −1 . Electrophysiological signals were analysed using Clampfit 9.2 (Axon Instruments) and IgorPro 6 software. General synthetic procedure To an isocyanate (1 mmol) in dry dichloromethane (10 ml) was added an amine (1 mmol), and the mixture was stirred at room temperature for 3–5 h. After dilution with dry dichloromethane (50 ml), malonyl chloride (1.1 mmol) was added dropwise under vigorous stirring at room temperature for 5 min. The resulting pale yellow solution was stirred for an additional 1 h and concentrated at reduced pressure to a small volume. The resultant reaction mixture was purified by flash chromatography on 50 g of silica gel in a column (20 mm internal diameter) using 20–33% ethyl acetate in hexanes to give analytically pure compounds (20–90% yield). Compound characterization data are shown in Supplementary Method S3 . Crystal structure acquisition A colourless plate crystal of 8 having approximate dimensions of 0.37×0.16×0.04 mm was mounted using oil (Infineum V8512) on a glass fibre. All measurements were made on a Bruker APEX-II CCD detector with MX optics monochromated CuK\α radiation and processed using SAINTPLUS from Bruker. The data were collected at a temperature of 100 K with a theta range for data collection of 6.16–67.32°. Data were collected in 0.5° oscillations with 5 s exposures. The crystal-to-detector distance was 40.00 mm. Accession codes: The X-ray crystallographic coordinates for structures reported in this Article have been deposited at the Cambridge Crystallographic Data Centre (CCDC), under deposition number CCDC 899840. These data can be obtained free of charge from The Cambridge Crystallographic Data Centre via http://www.ccdc.cam.ac.uk/data_request/cif . How to cite this article: Kang, S. et al . Ca V 1.3-selective L-type calcium channel antagonists as potential new therapeutics for Parkinson's disease. Nat. Commun. 3:1146 doi: 10.1038/ncomms2149 (2012).